Selective reduction and homologation of carbon monoxide by organometallic iron complexes Carbon monoxide is a key C 1 feedstock for the industrial production of hydrocarbons, where it is used to make millions of tonnes of chemicals, fuels, and solvents per annum. Many transition metal complexes can coordinate CO, but the formation of new C−C bonds in well-defined compounds from the scission and subsequent coupling of two or more CO moieties at a transition metal centre remains a challenge. Herein, we report the use of low-coordinate iron(II) complexes for the selective scission and homologation of CO affording unusual squaraines and iron carboxylates at ambient temperature and pressure. A modification of the ligand framework allows for the isolation and structural characterisation of a proposed metallacyclic Fe(II) carbene intermediate. These results indicate that, with the appropriate choice of supporting ligands, it is possible to cleave and homologate carbon monoxide under mild conditions using an abundant and environmentally benign low-coordinate, first row transition metal. CO activation is a critical reaction in organometallic chemistry, where it can be used to form valuable organic compounds through both homogeneous and heterogeneous catalytic transformations. These include carbonylation, hydroformylation, polymerisation, hydroesterification, and syngas conversion [1] , [2] , [3] . Early investigations of homogeneously catalysed CO hydrogenation and oligomerisation required the use of prohibitively high temperatures and pressures, affording only simple oligomers in low yield [3] . This can be improved somewhat through the use of additives such as Lewis acids, Lewis bases, or Brønsted acids. The study of model systems such as [(η 5 -C 5 H 5 )Fe(CO) 3 ] + , aided by the addition of reducing agents and Lewis base, allowed the fundamental steps in these processes to be elucidated [4] , [5] , [6] , [7] . Such electron-rich systems, however, are unable to undergo facile carbonylation; requiring borohydrides for carbonyl reduction and the use of relatively strong electrophiles to release homologated products [3] . The literature is replete with examples of migratory insertion of CO into M−C bonds. Of particular note is the reduction of coordinated CO by insertion into M–H and M–alkyl bonds, resulting in formyl or acyl species respectively, where the formal oxidation of the ligand permits the reduction of CO [7] , [8] . Acyl intermediates can act as a precursor for the formation of C 2 species and higher oligomers. Alternatively, the coupling of CO with carbenes forming η 2 -ketene complexes provides another route to C–C bond formation [9] , [10] . More interesting still is the chemistry reported for several zirconium complexes, where CO is not only inserted into the M−H bond, but the reductive coupling of two or more CO molecules has been reported [11] , [12] , [13] , [14] . Although the reductive coupling of CO remains unusual, there are a number of examples from across the periodic table, including the p-block [15] , [16] , d-block [12] , [17] , [18] , [19] , [20] , [21] , [22] , [23] , [24] , [25] , [26] and f-block [27] , [28] , [29] , [30] , [31] , [32] , [33] , [34] . The scission and homologation of CO to generate synthetically useful compounds under mild conditions remains a significant challenge. The C≡O bond is the strongest bond in chemistry (CO bond dissociation energy = 1076 kJ mol ‒1 ) [35] and the complete cleavage of CO requires six electrons for reduction. However, complexes of the d-block and f-block elements have been shown to form a range of compounds through mechanisms involving the complete scission of C≡O followed by homologation [12] , [36] , [37] , [38] , [39] , [40] , [41] , [42] , [43] , [44] . Previous work on C 4 ring formation via CO activation has yielded squarates (C 4 O 4 2‒ ) from uranium complexes, which does not require the scission of C≡O bonds [27] . The reductive coupling and cleavage of CO is unknown for low-coordinate iron species [45] , [46] , with early studies indicating that CO coupling was promoted by high-coordinate transition metal complexes [47] . Furthermore, previously reported reactions between transition metal m -terphenyl complexes and CO afforded only insertion products such as acyl complexes [48] , [49] and sterically encumbered ketones [50] . Herein, we report the complete scission of C≡O by low-coordinate Fe II complexes at ambient temperature and pressure, accompanied by the formal oxidation of the terphenyl ligand, affording unusual 1,3-squaraines through C–C coupling reactions with concomitant formation of Fe II carboxylate complexes and Fe(CO) 5 . These squaraine species feature broken conjugation (resulting in atypical electronic and bonding properties) and represent the first examples of C 4 ring formation from CO involving complete cleavage of the C≡O bond. Reactions between iron diaryl complexes and carbon monoxide Exposure of a toluene solution of 1 Mes [51] or 1 Xyl to excess CO at ambient temperature and pressure (Fig. 1a ) results in an immediate colour change from yellow to red; further stirring for 6 days ( 1 Mes ) or 36 h ( 1 Xyl ) under a CO atmosphere forms a dark red suspension. Recrystallisation from hexane at −30 °C ( 1 Mes ) or the layering of pentane onto a toluene solution at room temperature ( 1 Xyl ) affords red crystals of the squaraine molecules 2 Mes and 2 Xyl suitable for single crystal X-ray diffraction. The molecular structures of 2 Mes and 2 Xyl feature a central four-membered ring {C 4 O 2 } with m -terphenyl substituents bound to each side (Fig. 1b and Supplementary Fig. 2 ). 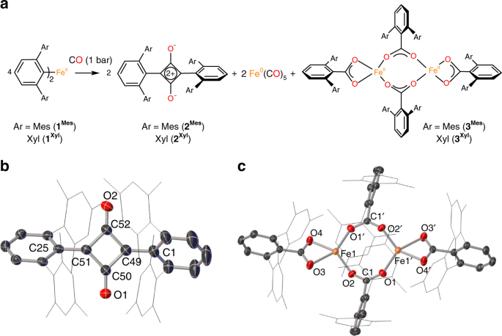Fig. 1 The reductive coupling and functionalisation of CO by iron(II) diaryls1Mesand1Xyl.aGeneral scheme for the reaction between CO and iron(II) diaryls1Mesor1Xyl.bThe molecular structure of2Meswith anisotropic displacement ellipsoids set at 50% probability. Mesityl groups shown as wireframe, hydrogen atoms and one molecule of hexane solvent are omitted for clarity.cThe molecular structure of3Meswith anisotropic displacement ellipsoids set at 50% probability. Mesityl groups shown as wireframe and hydrogen atoms have been omitted for clarity. Selected bond distances (Å) and angles (°) for3Mes: Fe1–O1 1.9736(11), Fe1–O2 1.9357(11), Fe1–O3 2.1909(13), Fe1–O4 2.0232(12), O1–Fe1–O2 109.30(5), O3–Fe1–O4 61.77(5) Selected bond distances and angles for 2 Mes and 2 Xyl can be found in Table 1 . Fig. 1 The reductive coupling and functionalisation of CO by iron(II) diaryls 1 Mes and 1 Xyl . a General scheme for the reaction between CO and iron(II) diaryls 1 Mes or 1 Xyl . b The molecular structure of 2 Mes with anisotropic displacement ellipsoids set at 50% probability. Mesityl groups shown as wireframe, hydrogen atoms and one molecule of hexane solvent are omitted for clarity. c The molecular structure of 3 Mes with anisotropic displacement ellipsoids set at 50% probability. Mesityl groups shown as wireframe and hydrogen atoms have been omitted for clarity. Selected bond distances (Å) and angles (°) for 3 Mes : Fe1–O1 1.9736(11), Fe1–O2 1.9357(11), Fe1–O3 2.1909(13), Fe1–O4 2.0232(12), O1–Fe1–O2 109.30(5), O3–Fe1–O4 61.77(5) Full size image Table 1 Selected experimental (X-ray, 2 Mes and 2 Xyl ) and calculated (DFT optimised, 2a ) bond distances (Å) and angles (°) Full size table In contrast to other aryl-substituted squaraines, where the aryl rings typically lie in-plane with the C 4 O 2 ring to maximise conjugation (average dihedral angle between aryl ring and C 4 O 2 ring = 1.24°) [52] , the aromatic rings in 2 Mes and 2 Xyl are twisted out of plane with the central ring [ 2 Mes : 56.38(13)° and 51.71(11)°, 2 Xyl : 50.93(5)°]. This is likely due to the steric demands of the terphenyl substituents. The C–O bond lengths in these compounds are also shorter than those found in typical squaraines [ 2 Mes : O1‒C50 1.214(3) Å, C52‒O2 1.218(3) Å; 2 Xyl : O1‒C14 1.212(2) Å; average squaraine C–O bond length = 1.24 Å] [52] . This is indicative of greater C–O double bond character, which is likely due to reduced conjugation with the aromatic substituents. The Fe II carboxylate complexes 3 Mes and 3 Xyl (Fig. 1a ) are also formed in the reaction of 1 Mes or 1 Xyl with CO and their solid-state structures have been confirmed by X-ray crystallography. The geometry around these Fe centres (Fig. 1c and Supplementary Fig. 3 ) is a distorted seesaw [τ 4 = 0.57 ( 3 Mes ) and 0.54 ( 3 Xyl )] [53] , and results from the coordination of Fe by one terminal and two bridging carboxylate ligands in which the angles between the FeO 2 planes defined by O1′‒Fe1‒O2 and O3‒Fe1–O4 are 46.634(3)° and 40.94(13)° for 3 Mes and 3 Xyl , respectively. When one considers the balanced reaction scheme (Fig. 1a ), it is important to mention that the formal oxidation of the ligand is essential for the reduction of CO. In the overall reaction, there is a net reduction of iron by four electrons and a net reduction of CO by four electrons, giving a total net reduction of eight electrons from the oxidation of the aryl ligands. The reaction between 1 Mes and CO was found to be near-quantitative, as determined by NMR integration against an internal standard (see Supplementary Methods). However, isolated yields were low due to difficulties in separating 2 Mes from 3 Mes , as the compounds have similar solubility. Analogous attempts to quantify the reaction between 1 Xyl and CO by NMR spectroscopy were hampered by the precipitation of 2 Xyl /3 Xyl mixtures (see Supplementary Methods ). Squaraine 2 Mes has been characterised by 1 H and 13 C{ 1 H} NMR, IR and UV/Vis spectroscopies and by mass spectrometry. The 13 C{ 1 H} NMR spectrum [C 6 D 6 solution, Supplementary Fig. 5 (a)] contains peaks at δ C 269.7 and 177.3 ppm, corresponding to the carbonyl (O C C) and the terphenyl-bound carbons in the C 4 O 2 ring, respectively. The assignment of the chemical shift at 269.7 ppm to the remarkably deshielded carbonyl (O C C) of 2 Mes is confirmed by 1 H, 13 C-HMBC NMR spectroscopy [Supplementary Fig. 5 (b)]. This, again, most likely results from the steric demands of the pendant terphenyl groups forcing the aryl ring to twist out-of-plane with the C 4 O 2 ring, which results in less charge delocalisation. In addition, most squaraines possess a donor–acceptor–donor (D–A–D) configuration where charge is delocalised into the C 4 O 2 ring [54] , [55] , [56] , [57] , a feature which is absent here. For example, squaraines with N , N -diarylanilino substituents display 13 C{ 1 H} NMR peaks for the C 4 O 2 ring in the range of 160 to 185 ppm [58] . Similarly, the solution IR spectrum of 2 Mes in toluene possesses a C–O stretch at 1673 cm −1 (Supplementary Fig. 12 ), which is at a higher frequency than typical squaraines (range 1594–1633 cm ‒1 ) [54] , [56] , [59] . To gain insight into the structures of 2 Mes and 2 Xyl , gas-phase DFT geometry optimisations were performed on a model compound of 2 Mes and 2 Xyl ( 2a ), in which the flanking mesityl and xylyl substituents were replaced by phenyl groups. Calculations for 2a give geometrical parameters (Table 1 ) that are in good agreement with those of the experimentally determined structures of 2 Mes and 2 Xyl . Additionally, 2a features a non-planar core with a dihedral angle between C 4 O 2 ring and the aryl substituent of 47.38°, slightly smaller than those observed in 2 Mes and 2 Xyl [ 2 Mes : 56.38(13)° and 51.71(11)°, 2 Xyl : 50.93(5)°]. Squaraines have previously been isolated in the singlet ground state [60] and RASSCF calculations [61] indicate that closed-shell singlet is the predominant electronic configuration for 2a (see Supplementary Methods ). The calculated C‒O stretching frequency for 2a is 1720 cm −1 (scaled by 0.95), which is higher than that found experimentally [1673 cm −1 ( 2 Mes ) and 1695 cm −1 ( 2 Xyl )]. This is not unexpected, as it has been documented that calculations which assume a harmonic approximation may overestimate IR stretching frequencies [38] . Labelling studies and mechanistic investigations Reactions between 1 Mes or 1 Xyl and 13 CO show that the squaraine molecules ( 2 Mes and 2 Xyl ) incorporate four C atoms [C49 to C52 ( 2 Mes ) and C13 to C14 ( 2 Xyl )] from CO into the central C 4 O 2 ring. This requires complete C≡O bond cleavage and the formation of new C–C bonds, which is significant as the reactions between CO and 1 Mes or 1 Xyl take place under ambient conditions in the absence of an external reducing agent. The reaction between 1 Mes and 13 CO generates 2 Mes - 13 C , where the 13 C{ 1 H} NMR spectrum displays triplet resonances for the central 13 C 4 O 2 ring [ δ C 269.7 ppm (t, 1 J (C,C) = 45 Hz, C O), 177.3 ppm (t, 1 J (C,C) = 45 Hz, C CO)]. Furthermore, 13 C, 13 C-COSY NMR (Supplementary Fig. 6 ) shows a correlation between these C atoms, providing further evidence that the four carbon atoms of the central 13 C 4 O 2 ring must originate from 13 CO. The solution IR spectrum of 2 Mes - 13 C displays an absorption at 1638 cm −1 (Fig. 2c ). DFT calculations of 2a- 13 C predict a vibrational frequency (1675 cm ‒1 ) that is 37 cm −1 higher than that determined experimentally (Supplementary Table 3 ). 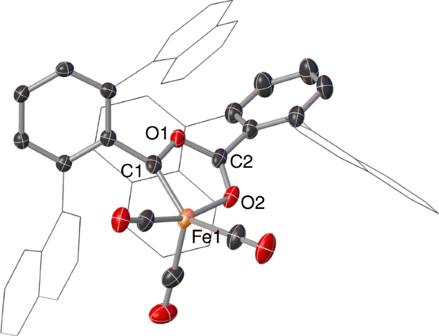Fig. 3 Molecular structure of4. Structure of4with anisotropic displacement ellipsoids set at 50% probability. Naphthyl groups shown as wireframe, hydrogen atoms and one molecule of Et2O solvent have been omitted for clarity. Selected bond distances (Å) for4: Fe1–C1 1.840(3), Fe1–O2 1.9572(18), Fe1–C3 1.830(3), Fe1–C4 1.753(3), Fe1–C5 1.849(3), C1–Fe1–O2 81.16(9) However, the ratio of the calculated frequencies ( 13 C/ 12 C = 0.974), compares well with that of the experimental values (0.979). Isolated samples of 2 Mes - 13 C contain a minor by-product that is observed as two doublets in the 13 C{ 1 H} NMR spectrum [ δ C 193.6 (d, 1 J (C,C) = 108 Hz, C=C=O), 24.8 (d, 1 J (C,C) = 108 Hz, C=C=O), see Supplementary Fig. 7 ], which are attributed to a ketene- or ketenyl-type intermediate in the formation of 2 Mes and 2 Xyl [37] , [62] . Fig. 2 IR spectroscopic monitoring of the reaction between 1 Mes and carbon monoxide. a IR spectra in toluene at room temperature obtained from the reaction of 1 Mes with CO; an aliquot was taken from the reaction mixture at the indicated times, dried under vacuum for ca. 1 h and dissolved in toluene. b Zoom of a between 1800 and 1550 cm –1 ; spectra recorded at 6 days and 9 days. c IR spectra in toluene at room temperature obtained from the reaction of 1 Mes with 13 CO; an aliquot was taken from reaction mixture at the indicated times, dried under vacuum for ca. 1 h and dissolved in toluene Full size image To gain insight into the reaction between 1 Mes and CO, the progress of the reaction was monitored by IR (Fig. 2a, b ) and NMR spectroscopies. Initially, three new IR bands appeared 35 min after the addition of CO to the reaction mixture ( ν = 2097, 2050, 1978 cm −1 ). The band at 2097 cm −1 increased in intensity whilst the bands at 2050 and 1978 cm −1 decreased in intensity over the course of the reaction. The bands at 2050 and 1978 cm −1 are most likely associated with terminal Fe carbonyls [63] and occur in a similar range to those of the Fe II carbonyl species, (η 2 -2,6-Dipp 2 C 6 H 3 CO) 2 Fe(CO) 2 , ( ν = 2000, 1944 cm −1 ) [48] , whilst the band at 2097 cm −1 is consistent with a ketene or ketenyl species (C=C=O), which appear in the range 2080 to 2250 cm −1 [62] . The reaction between 1 Mes and 13 CO was also monitored by IR spectroscopy (Fig. 2c ) and features bands between 1638–2038 cm −1 , all of which are shifted with respect to those observed in the analogous reaction between 1 Mes and CO (Supplementary Table 1 ). Monitoring the reaction by 1 H and 13 C{ 1 H} NMR spectroscopy in C 6 D 6 shows the disappearance of the peaks associated with 1 Mes immediately after the addition of CO, followed by the appearance of 2 Mes and paramagnetically shifted peaks after 19 h. After 30 h crystals formed, which were determined to be a mixture of 2 Mes and 3 Mes by X-ray diffraction. The formation of Fe(CO) 5 was confirmed in the reaction between 1 Mes or 1 Xyl and CO by IR and NMR spectroscopy, with bands at 2024 and 1999 cm −1 (Supplementary Fig. 15 ) [64] , and a singlet at 211 ppm in the 13 C{ 1 H} NMR spectra. To investigate further the influence of the aryl substituents on the reaction of m -terphenyl iron(II) complexes with CO, a solution of (2,6-Naph 2 C 6 H 3 ) 2 Fe(THF) ( 1 Naph ; Naph = 1-C 10 H 7 ) in Et 2 O was exposed to CO. After stirring at room temperature overnight, the reaction was worked up to afford red crystals of the metallacyclic Fe II carbene (CO) 3 Fe[C(2,6-Naph 2 C 6 H 3 )OC(O)(2,6-Naph 2 C 6 H 3 )] ( 4 ) that were suitable for X-ray diffraction measurements (Fig. 3 ). The solid-state structure of 4 exhibits an Fe II centre in a distorted square-pyramidal environment (τ 5 = 0.37). Compound 4 displays complex (see Supplementary Discussion and Supplementary Fig. 8 ) diamagnetic 1 H and 13 C{ 1 H} NMR spectra (Supplementary Figs. 9 and 10 ) and could represent an isolable analogue of an intermediate species in the reaction of 1 Mes /1 Xyl with CO. Treating compound 4 with excess CO failed to yield any further reaction, even after prolonged heating (80 °C for 14 h, see Supplementary Methods ). Fig. 3 Molecular structure of 4 . Structure of 4 with anisotropic displacement ellipsoids set at 50% probability. Naphthyl groups shown as wireframe, hydrogen atoms and one molecule of Et 2 O solvent have been omitted for clarity. Selected bond distances (Å) for 4 : Fe1–C1 1.840(3), Fe1–O2 1.9572(18), Fe1–C3 1.830(3), Fe1–C4 1.753(3), Fe1–C5 1.849(3), C1–Fe1–O2 81.16(9) Full size image It is possible to propose a pathway for the formation of the squaraines ( 2 Mes and 2 Xyl ) and Fe carboxylates ( 3 Mes and 3 Xyl ) from 1 Mes and 1 Xyl (Fig. 4 ) that is consistent with all spectroscopic data and the observation of compound 4 . The proposed mechanism also accounts for the observation (from 13 C labelling) that all carbons in the C 4 O 2 ring derive from CO. Fig. 4 Proposed pathway for the conversion of the iron(II) diaryls 1 Mes , 1 Xyl and 1 Naph to 2 – 4 . Proposed mechanism for the reaction between 1 Mes , 1 Xyl , and 1 Naph and CO forming squaraines 2 Mes and 2 Xyl , carboxylate complexes 3 Mes and 3 Xyl and carbene complex 4 . In the case of Ar = naphthyl, D = complex 4 Full size image First, CO coordinates to the Fe II centre in the diaryl complexes A , followed by 1,1-migratory insertion of CO into the Fe−C σ-bonds of the two m -terphenyl ligands to form an acyl intermediate of the type B . A similar Fe II acyl complex has previously been observed in the reaction of (2,6-Dipp 2 C 6 H 3 ) 2 Fe with CO [48] , [49] . Compound B then undergoes intramolecular C−O bond formation via keto-carbene tautomerisation to the carbene intermediate C [65] , [66] . Attack of the carbonyl carbon by the CO − unit forms the Fe carbene intermediate ( D ) [65] , [66] , which is analogous to the Fe carbene complex 4 . Species D may then react with CO [44] , [62] , [67] , [68] , to produce a ketenyl complex, with concomitant CO bond scission between the carbene C and carboxylate O to form intermediate E . Species E then dimerises to form iron ketenyl carboxylate complex F , similar to those observed in the reaction of CO with low valent organolanthanide complexes [38] , [40] . The coordinated ketene units may then dimerise in a [2 + 2] cycloaddition reaction affording 2 Mes / 2 Xyl in an analogous manner to that for uncoordinated ketenes, which dimerise to form 1,3-cyclobutanediones [62] . The concomitant dimerisation of the Fe-carboxylate units in F form the diiron carboxylate complexes 3 Mes / 3 Xyl and liberate Fe(CO) 5 . Given the disparate reactivities of 1 Naph and 1 Xyl / 1 Mes on treatment with CO, the mechanism proposed in Fig. 4 was probed by DFT, focusing on the conversion of D to E (see Supplementary Methods ). For the xylyl substituted complex, the barrier to reaction (Δ ‡ G °) is +14.6 kcal mol ‒1 , with a favourable Δ r G ° of ‒15.6 kcal mol ‒1 . However, formation of the naphthyl substituted E has a larger energetic barrier (Δ ‡ G ° = 22.8 kcal mol ‒1 ) and is thermodynamically unfavourable (Δ r G ° = +19.6 kcal mol ‒1 ). This striking difference is attributed to greater steric repulsion in E Naph , where the CO ligands and ketene clash with the large naphthyl flanking groups (Supplementary Fig. 22 ). This result helps rationalise why 4 is an isolable complex, while the corresponding carbene is not observed in the reactions of 1 Mes and 1 Xyl with CO, and highlights how the reactivity of these systems is heavily dependent on the nature of the flanking aryl groups. This reactivity is rather remarkable when compared with other open shell iron(II) hydrocarbyls [45] , [46] and transition metal terphenyls [48] , [49] , [50] which, although they undergo carbon monoxide coordination and migration, do not cleave C≡O bonds. Presumably this is due to factors such as the overall ligand field strength, complex geometry, and steric effects, which we have shown (through theoretical calculations) are heavily dependent on the flanking aryl groups of the m -terphenyl ligands. The importance of steric effects in CO activation has been demonstrated previously [19] , [69] . Furthermore, our system contrasts with electron-rich systems such as the [(η 5 -C 5 H 5 )Fe(CO) 3 ] + model complex, which do not readily undergo carbonyl reduction and require the use of electrophiles to release homologated products [3] . Electrochemical investigations of squaraines The electrochemical properties of 2 Mes were investigated by cyclic voltammetry, which revealed a reversible reduction process at E 1/2 = ‒0.79 V vs Fc + /Fc (Supplementary Fig. 13 ). This is significantly more anodic than typical squaraines, which possess reduction processes in the range of ‒1.40 to ‒0.98 V vs Fc + /Fc [55] , [58] . The reduction process is localised principally on the C 4 O 2 ring in 2 Mes (vide infra) and the difference in reduction potential is consistent with this moiety being electron deficient due to decreased conjugation with the aromatic rings. In addition, 2 Mes displays an irreversible oxidation process at E p a = + 0.48 V vs Fc + /Fc (Supplementary Fig. 14 ). Monoanionic 2 Mes•‒ and 2 Mes•‒ - 13 C were prepared by the addition of Cp 2 Co (Cp = η 5 -C 5 H 5 ) to a solution of 2 Mes or 2 Mes - 13 C in CH 2 Cl 2 . The experimental X-band EPR spectra, along with the simulated spectra, are shown in Fig. 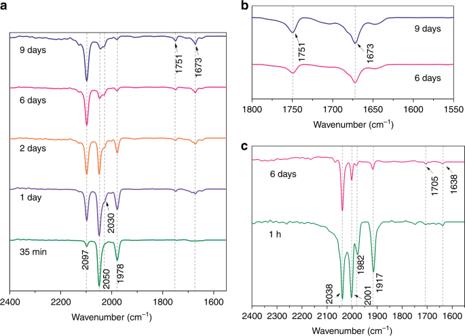5 . Fig. 2 IR spectroscopic monitoring of the reaction between1Mesand carbon monoxide.aIR spectra in toluene at room temperature obtained from the reaction of1Meswith CO; an aliquot was taken from the reaction mixture at the indicated times, dried under vacuum for ca. 1 h and dissolved in toluene.bZoom ofabetween 1800 and 1550 cm–1; spectra recorded at 6 days and 9 days.cIR spectra in toluene at room temperature obtained from the reaction of1Meswith13CO; an aliquot was taken from reaction mixture at the indicated times, dried under vacuum for ca. 1 h and dissolved in toluene The spectra show hyperfine couplings to 1 H and 13 C centres and may be simulated using the spin Hamiltonian parameters shown in Supplementary Table 2 . The room temperature X-band EPR spectrum of 2 Xyl•− in CH 2 Cl 2 solution (generated from the addition of Cp 2 Co to 2 Xyl ) is shown in Supplementary Fig. 19 , with simulation parameters in Supplementary Table 2 . 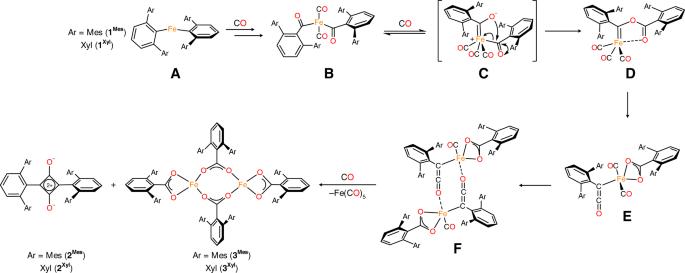Fig. 4 Proposed pathway for the conversion of the iron(II) diaryls1Mes,1Xyland1Naphto2–4. Proposed mechanism for the reaction between1Mes,1Xyl, and1Naphand CO forming squaraines2Mesand2Xyl, carboxylate complexes3Mesand3Xyland carbene complex4. In the case of Ar = naphthyl,D= complex4 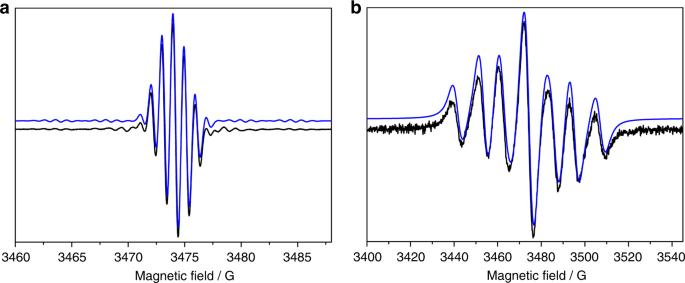Fig. 5 Spectroscopic investigations of2Meswith Cp2Co in CH2Cl2at room temperature.aExperimental X-band EPR spectrum of2Mes•‒(black trace) recorded as a fluid solution in CH2Cl2at room temperature. The simulated spectrum is given in blue and parameters used for the simulation are listed in Supplementary Table2.bExperimental X-band EPR spectrum of2Mes•‒-13C(black trace) recorded as a fluid solution in CH2Cl2at room temperature. The simulated spectrum is given in blue and parameters used for the simulation are listed in Supplementary Table2 Unrestricted DFT calculations of the hyperfine coupling constants of 2a •‒ (Supplementary Table 4 ) show a close correspondence with those derived from the EPR simulations of 2 Mes•‒ and are consistent with a spin density distribution (Supplementary Fig. 21 ) that lies across the central {(C 6 H 3 ) 2 C 4 O 2 } core with little delocalisation onto the flanking aryl substituents. Fig. 5 Spectroscopic investigations of 2 Mes with Cp 2 Co in CH 2 Cl 2 at room temperature. a Experimental X-band EPR spectrum of 2 Mes•‒ (black trace) recorded as a fluid solution in CH 2 Cl 2 at room temperature. The simulated spectrum is given in blue and parameters used for the simulation are listed in Supplementary Table 2 . b Experimental X-band EPR spectrum of 2 Mes•‒ - 13 C (black trace) recorded as a fluid solution in CH 2 Cl 2 at room temperature. The simulated spectrum is given in blue and parameters used for the simulation are listed in Supplementary Table 2 Full size image Two-coordinate iron(II) diaryl complexes promote the reductive cleavage and homologation of CO to yield {C 4 O 2 } species at room temperature and atmospheric pressure, converting C 1 feedstocks into useful organic molecules through a single first-row transition metal site. Unlike past work on C 4 ring formation through homologation, these reactions proceed via C≡O bond cleavage, and afford unusual squaraine species featuring broken conjugation. The observation of well-defined intermediates in this reaction, in addition to evidence from spectroscopy and isotopic labelling, allows us to rationalise the CO activation processes and propose a reasonable mechanism that is in-line with experimental observations. Furthermore, this investigation provides additional insight into CO activation by transition metals, which is of relevance to a vast array of industrially important catalytic processes. For synthetic details, analytical data, full descriptions of the methods and details of the computational calculations contained in this paper see Supplementary Information . For full synthetic procedures and analytical data for the compounds herein see Supplementary Methods . For a view of the single crystal X-ray structure for compounds 1 Xyl , 2 Xyl , 3 Xyl , 1 Naph see Supplementary Figs. 1 – 4 , respectively. For selected NMR spectra of the compounds in this article see Supplementary Figs. 5 – 7 and 9 – 11 . Cyclic voltammograms of 2 Mes are found in the Supplementary Figs. 13 and 14 . Additional IR spectra and reaction monitoring figures are found in Supplementary Figs 12 and 15 – 18 . EPR parameters for the experimental and simulated EPR spectra for 2 Mes·‒ , 2 Mes·‒13C and 2 Xyl·‒ are given in Supplementary Table 2 . Computational methods are outlined in the Supplementary Methods . Geometry-optimised co-ordinates of all computed structures are given in Supplementary Tables 5 – 13 .